Darwinian evolution in a translation-coupled RNA replication system within a cell-like compartment The ability to evolve is a key characteristic that distinguishes living things from non-living chemical compounds. The construction of an evolvable cell-like system entirely from non-living molecules has been a major challenge. Here we construct an evolvable artificial cell model from an assembly of biochemical molecules. The artificial cell model contains artificial genomic RNA that replicates through the translation of its encoded RNA replicase. We perform a long-term (600-generation) replication experiment using this system, in which mutations are spontaneously introduced into the RNA by replication error, and highly replicable mutants dominate the population according to Darwinian principles. During evolution, the genomic RNA gradually reinforces its interaction with the translated replicase, thereby acquiring competitiveness against selfish (parasitic) RNAs. This study provides the first experimental evidence that replicating systems can be developed through Darwinian evolution in a cell-like compartment, even in the presence of parasitic replicators. The construction of an artificial cell or model protocell is hypothesized to provide important insights into the emergence of life from an assembly of non-living molecules [1] , [2] , the basic principles that underlie biological functions [3] , [4] , [5] and the production of new technology [6] , [7] . To date, several cellular functions have been reconstructed using simple compounds, such as fatty acids, that may have existed during the prebiotic era [8] , [9] , [10] , [11] , [12] . Using other approaches, including the semi-synthetic approach [13] and the supramolecular approach [13] , various cellular functions have been reconstituted from purified biological polymers, such as proteins and RNA, in either lipid vesicles or water-in-oil emulsions to determine the conditions sufficient for achieving the target biological functions [14] , [15] , [16] , [17] , [18] . However, the creation of an artificial cell that harbours the same level of evolutionary ability as natural organisms remains a major challenge. The evolution of living organisms is a result of the error-prone replication processes of genetic material, either DNA or RNA, by the replication enzyme translated from its own information. To date, several replication systems have been constructed either from various sets of RNA and proteins [19] , [20] or from RNA ribozymes only [21] , [22] , although these replication systems lack the process by which the genetic information is translated into proteins. To construct an artificial system that replicates in the same manner as natural organisms, through the translation of a replication enzyme, we combined an artificial genomic RNA that encodes an RNA-dependent RNA polymerase, the Qβ replicase, with a reconstituted translation system [23] , [24] . In this translation-coupled RNA replication (TcRR) system, the genomic plus-strand RNA (2,125 nucleotides) replicates using an RNA replicase translated from its own sequence via the synthesis of the complementary minus-strand (Genomic RNA replication, Fig. 1a ). The TcRR requires a cell-like compartment to ensure interaction between the translated replicase and the original genomic RNA. In this study, we encapsulated the TcRR system into a microscale 1–6 μm cell-like compartment, a water-in-oil emulsion [25] , [26] . 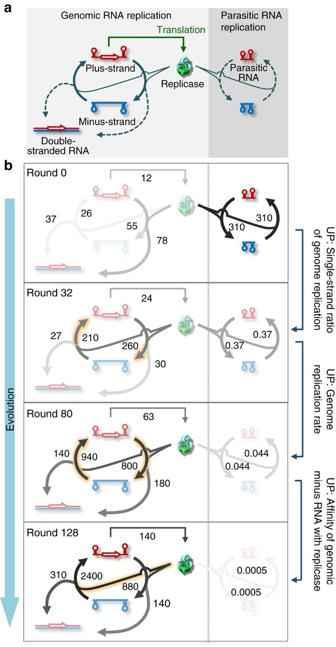Figure 1: A reaction network in a TcRR system. (a) Reaction scheme. The TcRR system is composed of genomic plus-strand RNA (2,125 nucleotides) encoding the catalytic β-subunit of Qβ RNA replicase and a purified translation system. The translated replicase replicates the original plus-strand RNA via complementary minus-strand RNA synthesis, during which the double-stranded RNA is produced via hybridization between the template and the newly synthesized strand. A parasitic RNA replicates and competes with the genomic RNA for the replicase. (b) The transition of reaction flow through evolution. The amount of reaction flow was simulated using the parameters shown inTable 1(initially, 100 nM plus-strand and 10 fM parasitic RNA). The intensity of the colour of the arrows and molecules roughly represents the quantities in the reaction. The absolute values are shown next to the arrows (nM h−1). Processes that were governed by the significantly changed parameters are highlighted in orange. Figure 1: A reaction network in a TcRR system. ( a ) Reaction scheme. The TcRR system is composed of genomic plus-strand RNA (2,125 nucleotides) encoding the catalytic β-subunit of Qβ RNA replicase and a purified translation system. The translated replicase replicates the original plus-strand RNA via complementary minus-strand RNA synthesis, during which the double-stranded RNA is produced via hybridization between the template and the newly synthesized strand. A parasitic RNA replicates and competes with the genomic RNA for the replicase. ( b ) The transition of reaction flow through evolution. The amount of reaction flow was simulated using the parameters shown in Table 1 (initially, 100 nM plus-strand and 10 fM parasitic RNA). The intensity of the colour of the arrows and molecules roughly represents the quantities in the reaction. The absolute values are shown next to the arrows (nM h −1 ). Processes that were governed by the significantly changed parameters are highlighted in orange. Full size image Translation coupling increases the complexity of the replication scheme; therefore, the TcRR system becomes vulnerable to selfish or parasitic RNAs, which are continuously generated from genomic RNA by the deletion of the internal replicase-encoding region, while retaining the terminal region for replicase recognition. These small RNAs are selfish and parasitic in that they do not produce replicase but replicate rapidly because of their small size (typically 222 nucleotides), utilizing the already existing replicase, until genome replication is competitively inhibited (parasitic RNA replication in Fig. 1a ) [27] . The genomic RNA must overcome the parasitic RNA to recursively replicate in the TcRR system. In the present study, we perform a long-term TcRR experiment in the manual fusion-division cycle of a cell-like compartment and find that genomic RNA can spontaneously evolve according to Darwinian principles and overcome the parasitic RNA through evolution. Long-term TcRR experiment increases replication ability We first performed a long-term TcRR experiment under conditions in which the RNA amplification was assisted by reverse transcription and PCR (RT-PCR) because of the inefficient replication during the initial stage ( Fig. 2a ). The plus-strand RNA (0.1 nM) was encapsulated with the purified translation system in a water-in-oil emulsion with a droplet diameter of 1–6 μm ( Supplementary Fig. S1 ); ~1 in 10 water droplets was expected to contain a single plus-strand RNA molecule. After incubation at 37 °C for 2 h to allow for RNA replication, we recovered and amplified the minus-strand RNA by RT-PCR and converted the complementary DNA into plus-strand RNA via in vitro transcription (IVT). The plus-strand was then re-encapsulated into the emulsion for the next round of replication cycle. This process was repeated 32 times, and mutations occurred via replication errors during each round (approximately one mutation per RNA per round, Supplementary Table S1 ). If a mutant RNA appeared with a greater ability to replicate, that RNA was expected to become dominant, increasing the average replication ability of the entire RNA population. In fact, the average fold replication (the ratio of the plus-strand concentration after replication to that before replication) was ~1.2-fold in round 1 and gradually increased to 30-fold in round 32 ( Fig. 2c ). No increase in the replication ability occurred in the control experiments without compartmentalization ( Fig. 3 ). 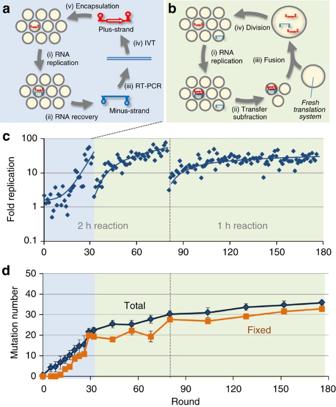Figure 2: Increased replication ability and mutation accumulation in a TcRR experiment. (a) The TcRR cycle method with RNA amplification (rounds 1–32). After (i) RNA replication in the emulsion, (ii) the synthesized minus-strand RNA was recovered and (iii) amplified by reverse transcription followed by PCR (RT-PCR). (iv) The resulting cDNA was converted to plus-strand RNA byin vitrotranscription (IVT) and then (v) re-encapsulated with the translation system in the emulsion for the next round of replication. (b) The simplified TcRR cycle method (rounds 33–176). After (i) RNA replication for 2 h (rounds 33–80) or 1 h (rounds 81–176), (ii) a subfraction of the emulsion was transferred and (iii) directly fused with a large droplet containing fresh translation system components by vigorous mixing; (iv) the droplet was then divided into droplets of the original size for the next round of replication. (c) The average fold replication of the plus-strand RNA population in the RNA replication step. The vertical dashed line represents the round at which the incubation time was shortened from 2 h to 1 h. (d) Mutation number. The sequences of 10–15 clones of plus-strand RNA were analysed at each round. The average number of total mutations (Total) and fixed mutations (Fixed) per RNA is plotted. Figure 2: Increased replication ability and mutation accumulation in a TcRR experiment. ( a ) The TcRR cycle method with RNA amplification (rounds 1–32). After (i) RNA replication in the emulsion, (ii) the synthesized minus-strand RNA was recovered and (iii) amplified by reverse transcription followed by PCR (RT-PCR). (iv) The resulting cDNA was converted to plus-strand RNA by in vitro transcription (IVT) and then (v) re-encapsulated with the translation system in the emulsion for the next round of replication. ( b ) The simplified TcRR cycle method (rounds 33–176). After (i) RNA replication for 2 h (rounds 33–80) or 1 h (rounds 81–176), (ii) a subfraction of the emulsion was transferred and (iii) directly fused with a large droplet containing fresh translation system components by vigorous mixing; (iv) the droplet was then divided into droplets of the original size for the next round of replication. ( c ) The average fold replication of the plus-strand RNA population in the RNA replication step. The vertical dashed line represents the round at which the incubation time was shortened from 2 h to 1 h. ( d ) Mutation number. The sequences of 10–15 clones of plus-strand RNA were analysed at each round. The average number of total mutations (Total) and fixed mutations (Fixed) per RNA is plotted. 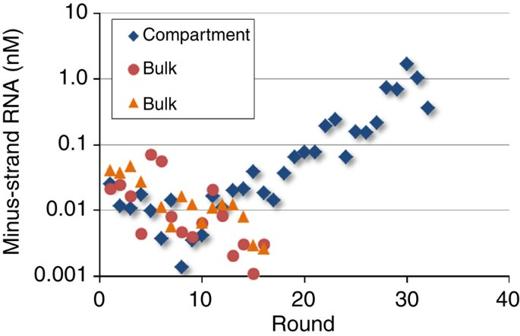Figure 3: No increase in the replication ability in the control TcRR cycles without compartmentalization. Two independent serial TcRR cycles were performed using the method represented inFig. 2a, without compartmentalization (Bulk); in these cycles, the initial plus-strand concentration was 1 nM, corresponding to the effective plus-strand concentration in the experiment with compartmentalization. The figure shows the average minus-strand RNA concentration after RNA replication. In both experiments, the minus-strand RNA gradually decreased and was no longer recovered after round 17. For comparison, the result of a TcRR cycle with compartmentalization (the same experiment represented inFig. 2) is also plotted (Compartment). Full size image Figure 3: No increase in the replication ability in the control TcRR cycles without compartmentalization. Two independent serial TcRR cycles were performed using the method represented in Fig. 2a , without compartmentalization (Bulk); in these cycles, the initial plus-strand concentration was 1 nM, corresponding to the effective plus-strand concentration in the experiment with compartmentalization. The figure shows the average minus-strand RNA concentration after RNA replication. In both experiments, the minus-strand RNA gradually decreased and was no longer recovered after round 17. For comparison, the result of a TcRR cycle with compartmentalization (the same experiment represented in Fig. 2 ) is also plotted (Compartment). Full size image As the replication ability improved, we simplified the TcRR cycle by eliminating the RT-PCR and IVT steps ( Fig. 2b ). After RNA replication, a subfraction of the droplets was transferred and directly fused by vigorous mixing with droplets that contained a fresh translation system. The resulting larger droplets were reduced to their original size via filtration for the next round of replication. Using the RNA population present after round 32, we repeated this process for another 48 rounds (rounds 33–80). During this time, the initial concentration of the plus-strand RNA was kept below 0.1 nM by adjusting the volume of the fused droplets ( Supplementary Fig. S2 ). The average replication, which decreased to twofold at round 33 because of the change in the process (see below for details), increased again to ~30-fold by round 80 ( Fig. 2c ). We then decreased the incubation time from 2 h to 1 h for an additional 96 rounds (rounds 81–176). The average replication at round 81 decreased to approximately fivefold before gradually increasing again. Through all the long-term replication processes, the genomic RNA replicated ~2 600 -fold, corresponding to 600 generations. The average fold replication decreased from ~30-fold to 2-fold at the transition from round 32 to 33 ( Fig. 2c ). This decrease is explained by the effect of omitting RNA labelling after round 32. Before round 32 ( Fig. 2a ), the plus-strand RNA was labelled with α-S GTP in the IVT to selectively degrade the initial plus-strand after RNA replication for selective recovery of newly synthesized RNA (see Methods), whereas the plus-strand was not labelled after round 32. The omission of labelling may have affected RNA folding, resulting in a decrease in the replication ability of the RNA at round 32 after it had adapted under the labelled condition. Mutations are fixed in the genomic RNA To test whether evolution led to the gradual increase in the replication ability ( Fig. 2c ), we analysed sequences of 10–15 RNA clones during each round. The average number of mutations per clone increased by ~0.7 per round and 0.1 per round before and after round 32, respectively ( Fig. 2d , total). The higher rate before round 32 resulted from the additional mutations that occurred during the RT-PCR and IVT processes. We defined the mutations observed in more than half of the analysed clones as ‘fixed.’ These fixed mutations increased intermittently ( Fig. 2d , fixed) and ultimately reached a total of 38 mutations, which included 34 point mutations, 1 insertion and 3 deletions ( Supplementary Table S2 ). These results (the increased replication ability, or fitness, and the successive fixation of the mutations) provide evidence of RNA evolution according to Darwinian principles. Each of the fixed mutations increased in frequency throughout the population with varying rates and dynamics ( Fig. 4 ). Some mutations (for example, numbers 8 and 9) increased slowly from round 8 to 29, but others (for example, numbers 16 and 17) were fixed rapidly within three rounds, presumably depending on the benefit each mutation offers for the RNA replication. The mutation (number 19) was fixed at round 29 but then disappeared at round 56 and was fixed again at round 80, suggesting the effect of clonal interference [28] . As the population size in the long-term TcRR experiment is ~10 7 –10 10 , mutations should rarely be fixed by genetic drift in 180 rounds [29] . Hence, each example of fixation dynamics is expected to contain at least one beneficial mutation. In addition, the deletion of 29 amino-acid residues at the C terminus of the replicase subunit (number 32) exactly matches the deleted region that has been reported to improve the replicase activity at the cost of template specificity [30] . 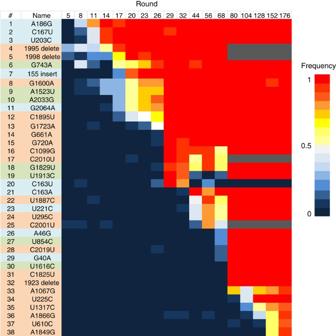Figure 4: Varying fixation dynamics of the mutations. The frequency of each mutation in the analysed clones is represented as a heat map. The grey colour indicates mutation regions that were lost in the large deletion that occurred in round 80 (number 32). Figure 4: Varying fixation dynamics of the mutations. The frequency of each mutation in the analysed clones is represented as a heat map. The grey colour indicates mutation regions that were lost in the large deletion that occurred in round 80 (number 32). Full size image Evolved RNAs are competent against the parasitic RNA To investigate changes in the reaction network between the genomic RNA, the translated replicase and the parasitic RNA via evolution, we analysed the biochemical properties of four RNA clones (one each from rounds 0, 32, 80 and 128; Supplementary Table S3 ). We first compared the TcRR kinetics for these clones in the emulsion ( Fig. 5a ). The replication of the original RNA (round 0) stopped within 0.5 h, and the final replication was less than twofold. As the rounds progressed (round 32, 80 and 128), the replication continued, and the RNA clone at round 128 replicated up to 200-fold after 4 h. In addition, the replication kinetics of round 32–128 became roughly exponential (that is, linear on a semi-logarithmic scale), suggesting that the replicated RNA recursively functioned as a template for the next replication cycle. 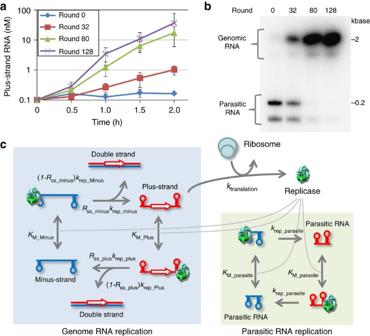Figure 5: Biochemical assessment of the genomic RNA clones chosen from rounds 0, 32, 80 and 128. (a) Time course data for TcRR of the plus-strand RNA clones. The TcRR reaction was performed with each plus-strand (0.1 nM) in the emulsion at 37 °C. At each time point, plus-strand concentrations in the droplets were measured. The error bars indicate the s.d. (n=2). (b) Competition experiment between genomic plus-strand RNA and a parasitic RNA. TcRR reactions were performed with each clone (50 nM) and a parasitic RNA (10 fM) without compartmentalization at 37 °C for 4 h. The replicated RNAs were detected by radioisotope labelling, followed by non-denatured polyacrylamide gel electrophoresis and autoradiography. The full image of the gel is shown in theSupplementary Fig. S9. (c) A kinetic model of TcRR. A Michaelis–Menten-type reaction was assumed for each RNA replication reaction (that is, the replication rate is represented askrep[RNA][Replicase]/(KM+[RNA]), wherekrepandKMare the maximum replication rate constant and the Michaelis constant, respectively). During replication, template RNA and newly synthesized RNA hybridize to form double-stranded RNA, a dead-end product of this system41. HereRssrepresents the fraction of synthesized RNA that is in the single-stranded form. For simplicity, the formation of double-stranded RNA of the parasitic RNA is neglected, and the same parameters are assumed for both complementary strands of the parasitic RNA. Double-stranded RNA formation by collision between the plus- and minus-strand RNA was omitted in this model because the rates are extremely small for all clones (Supplementary Fig. S8). Figure 5: Biochemical assessment of the genomic RNA clones chosen from rounds 0, 32, 80 and 128. ( a ) Time course data for TcRR of the plus-strand RNA clones. The TcRR reaction was performed with each plus-strand (0.1 nM) in the emulsion at 37 °C. At each time point, plus-strand concentrations in the droplets were measured. The error bars indicate the s.d. ( n =2). ( b ) Competition experiment between genomic plus-strand RNA and a parasitic RNA. TcRR reactions were performed with each clone (50 nM) and a parasitic RNA (10 fM) without compartmentalization at 37 °C for 4 h. The replicated RNAs were detected by radioisotope labelling, followed by non-denatured polyacrylamide gel electrophoresis and autoradiography. The full image of the gel is shown in the Supplementary Fig. S9 . ( c ) A kinetic model of TcRR. A Michaelis–Menten-type reaction was assumed for each RNA replication reaction (that is, the replication rate is represented as k rep [RNA][Replicase]/( K M +[RNA]), where k rep and K M are the maximum replication rate constant and the Michaelis constant, respectively). During replication, template RNA and newly synthesized RNA hybridize to form double-stranded RNA, a dead-end product of this system [41] . Here R ss represents the fraction of synthesized RNA that is in the single-stranded form. For simplicity, the formation of double-stranded RNA of the parasitic RNA is neglected, and the same parameters are assumed for both complementary strands of the parasitic RNA. Double-stranded RNA formation by collision between the plus- and minus-strand RNA was omitted in this model because the rates are extremely small for all clones ( Supplementary Fig. S8 ). Full size image We next performed a competition experiment in which the genomic plus-strand RNAs (50 nM) were mixed with a small quantity of parasitic RNA (10 fM) under bulk conditions (that is, without compartmentalization), and the replicated RNA was detected by the incorporation of radiolabelled UTP. Unlike the genomic RNA, the parasitic RNA replicated extensively with the original genomic RNA (round 0; Fig. 5b ). In contrast, the genomic RNA replicated more selectively as the rounds proceeded, indicating that it had higher competence against the parasitic RNA. A similar result was observed in an experiment without the addition of parasitic RNA when parasitic RNAs spontaneously developed from each genomic RNA molecule ( Supplementary Fig. S3A ). We also analysed the time course data of the TcRR reaction without compartmentalization ( Supplementary Fig. S3B ) and found that replication of the evolved clone (round 128) is prolonged, most probably because of competence against the parasitic RNA. To quantitatively evaluate these evolutionary changes, we measured the kinetic parameters of each genomic plus- and minus-strand RNA and the parasitic RNA as substrates for each purified replicase based on the kinetic model shown in Fig. 5c ( Table 1 ). Although the highly variable parameters were dependent on the round, most were related to the ability of genomic RNA to be replicated rather than the activity of the replicase enzyme ( Supplementary Fig. S4 ). In round 32, the single-strand ratios of the replication product for both the genomic plus- and minus-strands ( R ss_plus and R ss_minus ) increased from ~0.4 to 0.9 ( Table 1 ). In round 80, the genomic replication rate constant ( k rep_plus and k rep_minus ) increased approximately twofold. In round 128, the affinity between the replicase and the genomic minus-strand RNA (1/ K M_minus ) increased approximately sixfold. Table 1 Kinetic parameters of RNA clones at each round. Full size table To visualize the effect of the observed changes in the kinetic parameters on the replication reaction network, we evaluated the reaction flows in the TcRR via computer simulation ( Fig. 1b ). This simulation demonstrated that in round 0, most of the translated replicase was utilized to replicate the parasitic RNA and little was used for genomic replication, primarily leading to non-replicable double-stranded RNA. In round 32, more replicase was utilized for the genomic replication of the single-stranded form as reflected in the increased single-strand ratios ( R ss_plus and R ss_minus ). In round 80, even more replicase was utilized for the genomic replication as evidenced by the increase in the genomic replication rate constant ( k rep_plus and k rep_minus ). This trend was accelerated in round 128 because of the increased affinity between the replicase and the genomic minus-strand RNA (1/ K M_minus ). These results demonstrate that genomic RNA can acquire the ability to selectively replicate via evolution by reinforcing a cooperative relationship between the genomic RNA and a translated replicase. In this study, we constructed an artificial cell-like system in which the genomic RNA replicates as it does in natural organisms (that is, through translation of self-encoded replicase) and evolves according to Darwinian principles through the continuous fusion and division cycles of a cell-like compartment. The evolutionary self-improving ability differentiates this system from typical enzymatic reactions: the replication reaction repeats over many generations, and its replication reaction network is autonomously improved. This process occurs just as it has in natural organisms throughout their long evolutionary history. The evolvable artificial cell-like system constructed in this study represents a step towards the realization of an artificial cell with the same evolutionary potential as natural organisms. The evolutionary process of this system provides experimental insight into the following long-standing question regarding the origin of life: how can a primitive self-replication system be maintained by overcoming the appearance of selfish or parasitic replicators in prebiotic evolution [31] ? Theoretically, a self-replicating reaction network with a certain level of complexity, such as the hypercycle [32] , is easily destroyed by the appearance of parasitic replicators that selfishly replicate by exploiting the system’s resources [31] , [33] . These parasitic replicators often appear in artificial replication systems [34] , [35] . One possible solution for this problem is compartmentalization, which spatially restricts parasite propagation and allows group selection at the compartment level [32] , [33] , [36] . Szathmary and Demeter [36] have explicitly demonstrated the role of compartmentalization in the evolution of self-replication networks using the Stochastic Corrector Model, in which self-replication molecules are selected at the individual molecular level and the group level. Therefore, self-replication networks can be sustained and continue to evolve even in the presence of parasitic replicators. In the current study, we tested this model experimentally using a TcRR system and observed that compartmentalization sustains genomic replication for many generations ( Figs 2 and 3 ) and also allows the evolution of competitiveness against the parasitic RNA, supporting the validity of the Stochastic Corrector Model. This result provides experimental evidence that self-replication systems can be maintained and further developed through evolution in a cell-like compartment, even when they are surrounded by parasitic replicators. Does the evolution of the artificial system used in this study display features similar to those of natural organisms? In this work, we observed two evolutionary patterns that have also been observed in the experimental evolution of bacteria and viruses. First, the rate of increase in fold replication (that is, fitness) decreased as the experiment proceeded ( Fig. 2c ), a phenomenon that is known in bacterial evolution as ‘diminishing return [37] . Second, in contrast to the decreasing rate of increase in fitness, the accumulation of mutations continued at a relatively constant rate ( Fig. 2d ); this type of relationship has been characterized as a discrepancy between the tempo and the mode of evolution [38] , [39] . The mechanisms that produce these patterns in natural organisms are still unclear. The similarity of the patterns in the artificial replication system studied here to those found in nature indicates that these patterns do not depend on the complexity of natural cells but instead are common evolutionary features of asexual self-replicating systems composed of polynucleotides and proteins. The simpler reaction network of the in vitro system studied here provides a useful platform for discovering the mechanisms underlying these evolutionary patterns. This artificial cell-like system could also provide a useful platform to understand how an assembly of chemical molecules could become ‘alive’ through an evolutionary process. In principle, the genomic RNA obtained in this study has an unlimited potential to acquire new functions and develop a more complex network by encoding additional genes, including translation factors, that are currently supplied externally. Examining whether the genomic RNA could (with additional replication cycles) evolve to create a system that resembles a natural living organism or whether the evolution would be halted by other obstacles such as an error catastrophe [32] would be of interest. The TcRR provides a novel platform for the experimental investigation of evolutionary scenarios that may lead to the emergence of a ‘living state’ from the assembly of non-living molecules. Translation-coupled RNA replication Plus-strand RNA (0.1 nM) was mixed with the customized translation system ( Supplementary Table S4 ), and 10 μl of the mixture was dropped into 1 ml of buffer-saturated oil. The mixture of solution and oil was filtered through a multipore membrane (20 μm hydrophilic SPG pumping filter, SPG Techno, Japan) 40 times to prepare a 1–6-μm water-in-oil emulsion ( Supplementary Fig. S1 ). The buffer-saturated oil was prepared as follows. The freshly prepared oil phase (95% mineral oil (Sigma), 2% Span 80 (Wako, Japan) and 3% Tween 80 (Wako)) was immediately mixed vigorously for 30 s with 50–150 μl of saturation buffer per ml of oil and then incubated for 10 min at 37 °C. After centrifugation at 20 g at room temperature for 5 min, the upper oil phase was collected and used as the buffer-saturated oil phase. The composition of the saturation buffer was the same as that used in the cell-free translation system except that all proteins, RNAs and NTPs were omitted and the concentration of dithiothreitol was increased sixfold (to 36 mM). RNA measurement Plus-strand and minus-strand RNA concentrations were measured using RT-qPCR, as described in a previous study [27] . In some experiments, RNA was detected using autoradiography. In these experiments, cell-free translation mixtures containing [ 32 P]-UTP and reaction mixtures were subjected to 1% agarose gel electrophoresis in 1 × TBE (89 mM Tris-borate, 20 mM EDTA) at 4 °C to separate single-stranded and double-stranded forms of genomic RNA and to 8% polyacrylamide gel electrophoresis to separate genomic RNA from parasitic RNA. Electrophoresis was followed by fixation, drying and autoradiography as described in a previous study [27] . Methods for TcRR cycle Rounds 1–32: The original RNA (MDV(−)β(+)) was prepared by IVT with the exception of the addition of 1 mM Sp-GTP-α-S (BIOLOG Life Science Institute, Germany). The prepared template RNA was mixed with the cell-free translation system and encapsulated into an emulsion as described. After incubation at 37 °C for 2 h, water droplets were collected by centrifugation (20 g for 5 min at room temperature) and washed with diethyl ether as described previously [25] . At this stage, the plus-strand RNA concentration was measured using RT-qPCR to quantify the fold change in replication. The recovered water droplets were mixed with nine volumes of an iodine solution (10 mM iodine, 1 mM Tris-HCl (pH, 7.4)) and incubated for 5 min at 37 °C to degrade the initial plus-strand RNA [40] . This reaction was stopped by the addition of 10 mM dithiothreitol. The newly synthesized RNA was purified using an RNeasy column (QIAGEN). An aliquot (0.75 μl) of purified RNA was subjected to reverse transcription at 54 °C for 30 min using RTase (PrimeScript, Takara, Japan) and primer 1 according to the manufacturer’s instructions, followed by the addition of RNaseH and incubation for 20 min at 37 °C. An aliquot (<10%) of the solution was mixed with PCR solution (KOD-FX, Toyobo, Japan) and primers 1 and 2 to amplify the cDNA of the minus-strand RNA. The amplified cDNA (~2 kb) was purified using a DNA column (QIAGEN) and subjected to size selection by gel extraction (Invitrogen E-cell clone-well). After further purification on the QIAGEN DNA column, the cDNA was mixed with a DNA fragment harbouring terminal sequences prepared by PCR with primers 5 and 6 using pUC-MDV(−)β(+) as a template, and the full-length cDNAs were amplified using PCR (PrimeStar GXL, Takara) with primers 3 and 4. In this PCR reaction, the T7 promoter and terminal sequences that were lost during the previous PCR were attached to the cDNA. The resulting cDNA was digested with Sma I to determine the 3′-end and subjected to IVT with sp-α-S GTP as described above. The synthesized RNA was quantified by measuring its A 260 and used for the next round of the reaction. After round 32: The TcRR reaction was performed in an emulsion using plus-strand RNA at round 32. After the reaction, the average plus-strand RNA concentration in a water droplet was measured by RT-qPCR as described above. An aliquot of the emulsion (5–200 μl) was then mixed vigorously with 10 μl of cell-free translation solution using a vortex mixer for 30 s at maximum speed to mix all of the solution into droplets. The volume of the emulsion aliquot was adjusted based on the average plus-strand RNA concentration so that the final plus-strand RNA concentration was <0.1 nM. New oil phase (1 ml) was added, and the emulsion droplets were further reduced to their original size (1–6 μm) by filtration through a multipore membrane as described above. The resulting emulsion was then incubated for the next round of TcRR. Other methods including plasmids, primers, composition of the customized translation system are described in the Supplementary Methods . How to cite this article: Ichihashi, N. et al. Darwinian evolution in a translation-coupled RNA replication system within a cell-like compartment. Nat. Commun. 4:2494 doi: 10.1038/ncomms3494 (2013)